Pattern formation at multiple spatial scales drives the resilience of mussel bed ecosystems Self-organized complexity at multiple spatial scales is a distinctive characteristic of biological systems. Yet, little is known about how different self-organizing processes operating at different spatial scales interact to determine ecosystem functioning. Here we show that the interplay between self-organizing processes at individual and ecosystem level is a key determinant of the functioning and resilience of mussel beds. In mussel beds, self-organization generates spatial patterns at two characteristic spatial scales: small-scale net-shaped patterns due to behavioural aggregation of individuals, and large-scale banded patterns due to the interplay of between-mussel facilitation and resource depletion. Model analysis reveals that the interaction between these behavioural and ecosystem-level mechanisms increases mussel bed resilience, enables persistence under deteriorating conditions and makes them less prone to catastrophic collapse. Our analysis highlights that interactions between different forms of self-organization at multiple spatial scales may enhance the intrinsic ability of ecosystems to withstand both natural and human-induced disturbances. One of the most striking features of biological systems is the bewildering complexity at all levels of organization, ranging from the structure of organic molecules to the spatial organization of ecosystems. Untangling this biological complexity has developed into an exciting line of research, highly interdisciplinary in nature, and involving concepts that cut across many different fields [1] , [2] , [3] , [4] , [5] , [6] . Many ecosystems show patterns at multiple spatial scales, for example, in coral reefs [7] , savannahs [8] , [9] and seagrass ecosystems. Yet, because research questions and techniques often vary among different scales, there is a strong tendency to study the processes at these different scales separately [10] , [11] , [12] . For instance, some studies focus on the spatial patterns that result from the movement of individuals, for example, for shelter, improved mate choice or the sharing of information [5] , [13] , [14] , [15] , [16] , [17] . Other studies focus on large-scale ecosystem processes that create spatial variation in predation pressure, resource availability [8] , [12] , [18] , [19] , [20] and other environmental conditions [21] , [22] , [23] , [24] . However, little is known about how interactions between spatial pattern formation across different levels of organization, acting across different spatio-temporal scales, determine ecosystem functioning. Here we report on the interaction of behavioural and ecosystem-level mechanisms of pattern formation in self-organizing intertidal mussel beds. In mussel beds, patterns develop at two distinctly separate scales, in the form of large-scale banded patterns occurring at the ecosystem level ( Fig. 1a,b ), and small-scale net-shaped patterns at the scale of individual mussels ( Fig. 1c ). At the ecosystem level, pattern formation is driven by the interplay of two scale-dependent processes. Mussels compete for algae in the water column at large spatial scales (>1 metre) due to high flow rate of the tidal water, but facilitate each other at smaller scales (<1 metre) by locally accumulating sediment (a form of ecosystem engineering) within elevated hummocks of 1–4 metres width, which improves individual feeding efficiency [25] . This interplay between facilitation and competition explains the banded patterns occurring at the 5–10-metre scale [20] . At the smallest scale, individual mussels aggregate by means of density-dependent movement, actively moving into small clusters and out of larger ones, to form a reticulate network of clusters at ~15-cm intervals in which mussels attach to each other by means of byssal threads, thereby protecting each other against predation and dislodgement [13] , [14] , [26] , [27] . Both the large-scale banded patterns and the reticulate network of small-scale clusters result from a self-organization process, meaning that the patterns emerge from the interactions between the mussels, rather than being imposed by the landscape [1] . Pattern formation at the individual level is strikingly fast, occurring within days, while the large-scale banded patterns require many months to develop. Because of these two separate, yet interacting self-organizing processes, mussel beds provide a unique opportunity to investigate how pattern formation at different spatio-temporal scales affects the functioning of ecosystems. 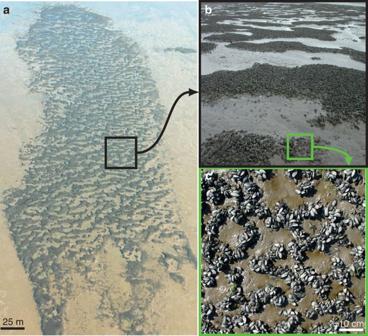Figure 1: Self-organized spatial patterns in a mussel bed at two spatial scales nested within one another. (a) Aerial view of a mussel bed on an intertidal flat, representing a width of ~200 metres. (b) Self-organized banded patterns within this bed, where the distance between successive mussel bands varies between 2 and 20 metres. (c) Small-scale clusters <20 cm in scale embedded within the mussel bands. Figure 1: Self-organized spatial patterns in a mussel bed at two spatial scales nested within one another. ( a ) Aerial view of a mussel bed on an intertidal flat, representing a width of ~200 metres. ( b ) Self-organized banded patterns within this bed, where the distance between successive mussel bands varies between 2 and 20 metres. ( c ) Small-scale clusters <20 cm in scale embedded within the mussel bands. Full size image The model We constructed an individual-based model (IBM) to study the development of mussel beds on intertidal flats. The model integrates small-scale aggregative movement of individual mussels with the large-scale processes of between-mussel facilitation and competition for algae. Movement of individual mussels is described by a random walk with an evenly distributed angle and a step size that obeys a statistical model derived in a previous paper [13] , where the movement step length of mussels follows an exponential distribution, h ( r , β )=(1/ β )exp(− r / β ), with parameter β =1/( p 0 + p 1 L 1 − p 2 L 2 ) (see Supplementary Table 1 for detailed interpretation and values of the parameters). This function expresses a scale-dependent effect of mussel density on individual movement, where L 1 and L 2 represent the density of other mussels in the neighbourhood at a scale of 1.5 and 6 cm, respectively. The large-scale population- and ecosystem-level processes are represented as partial differential equations (PDE), describing the local growth and mortality of mussels as determined by algal consumption, sediment accumulation and a density-dependent mortality rate [13] , [20] , [25] . Let A(x, y, t ) describe the algal concentration in the benthic boundary layer, M ( x, y, t ) the mussel density and S ( x, y, t ) the sediment elevation at location ( x, y ) and time t . This part of the model is then given by: where A up is the concentration of algae in the surface layer, f is the exchange rate between the benthic boundary layer and surface layer, c is the maximum consumption rate of algae by mussels, k s is the sediment level at which consumption is half maximal, g specifies the consumption of algae in the absence of sediment accumulation, e is the conversion efficiency of ingested algae to mussel density, d m is the maximum mortality rate of the mussels, k m is the mussel density at which mussel mortality is half maximal, k 1 is the deposition rate of sediment by mussels in the form of pseudofaeces and d s is the erosion rate of the sediment. Here, we assume that mussel mortality decreases with local mussel density because high, within-clump densities provide protection against predation and dislodgement [20] , [26] , [27] . Advection of algae is represented by the term V ∇ x A with velocity V . Local dispersion of sediment over the tidal flat is modelled by the diffusion term D s ∇ 2 S . We use the notation to express mussel movement behaviour, which is modelled explicitly as random walks of individual mussels (as described above). Local changes in mussel density are translated into the IBM model by random mortality of a fraction of the local individuals if local change is negative, or by random addition of new mussels if local change is positive. The detailed model formulation and simulation methods are described in the Methods section. The emergence of nested spatial patterning The model predicts the formation of nested spatial patterns in mussel beds, similar to the development of mussel beds under natural conditions ( Fig. 2 ). For comparison, we made photographs of mussel beds at various developmental stages, starting from a young mussel bed ~2 months after settlement to a strongly patterned bed of about 2 years of age. At first, behavioural aggregation through individual movement leads to the rapid development of clumped patterns at small spatial scales ( Fig. 2a,d ), while the bed remains relatively homogeneous at larger scales. As time progresses, the small-scale clumps develop into a reticulate network, while banded patterns develop at larger spatial scales due to differential growth and mortality. Increased sedimentation triggered by mussel feeding leads to the development of hummocks underneath mussel patches, which become raised from the seabed [25] ( Fig. 2b,e ). This leads in the long run to the development of a mature mussel bed with clear spatial patterns at two spatial scales ( Fig. 2c,f ): small-scale net-shaped patterns embedded in large-scale banded patterns. For all stages, the model results reveal a striking similarity between predicted patterns and those observed in the field, as is confirmed by spectral analysis of the spatial patterns revealing two dominant scales of 0.3 and 8.0 m, respectively ( Supplementary Fig. 1 ). This indicates that the model can well explain the emergence of nested patterns in mussel beds. 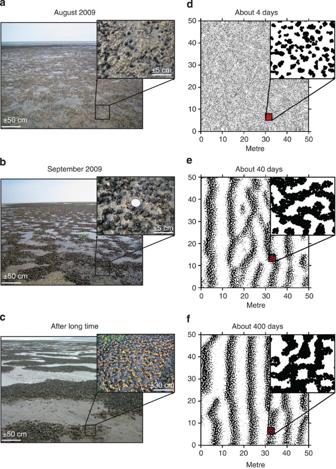Figure 2: Development of spatial patterns at two spatial scales within mussel beds. (a–c) Development of spatial patterns in the field. (a,b) A mussel bed at 2 months and 4 months after larval settlement in May/June 2009, on a tidal flat in the Wadden Sea (near De Cocksdorp, The Netherlands). (c) A mature, undisturbed mussel bed in the Menai strait (near Bangor, United Kingdom). (d–f) Model predictions of the development of self-organized spatial patterns at two spatial scales, nested within one another, in mussel beds of 4, 40 and 400 days old. The insets show a magnified view of the nested patterns. Figure 2: Development of spatial patterns at two spatial scales within mussel beds. ( a – c ) Development of spatial patterns in the field. ( a , b ) A mussel bed at 2 months and 4 months after larval settlement in May/June 2009, on a tidal flat in the Wadden Sea (near De Cocksdorp, The Netherlands). ( c ) A mature, undisturbed mussel bed in the Menai strait (near Bangor, United Kingdom). ( d – f ) Model predictions of the development of self-organized spatial patterns at two spatial scales, nested within one another, in mussel beds of 4, 40 and 400 days old. The insets show a magnified view of the nested patterns. Full size image Effect of spatial self-organization on ecosystem functioning We now use the model to investigate how this nested pattern formation affects the functioning of self-organized ecosystems. We used a full-factorial design to investigate the separate and combined effects of small-scale and large-scale self-organization, by switching off (1) the small-scale aggregative behaviour, (2) the large-scale ecosystem patterning and (3) both forms of spatial self-organization, and compared the predicted properties of the equilibria with that of the full self-organizing model. Small-scale aggregation was removed by switching off density-dependence of individual mussel movement (that is, h(r , β)= constant); large-scale spatial patterning was switched off by increasing the dispersion coefficient for sediment ( D s ) to a value outside the domain of pattern formation. Note that this method targets only the spatial dispersal in the model but none of the growth or mortality processes, making it possible to assess how the loss of self-organization affects ecosystem dynamics, an analysis that is rarely done. For each model variant, we determined changes in equilibrium mussel density as a function of algal concentration in the inflowing water ( A up ), which provides the major food source for mussel beds [20] . The results of the full-factorial model analysis reveal that the interplay between small-scale and large-scale self-organization has a strong impact on the resilience of this ecosystem. We first switched off all forms of self-organization, such that the mussels are homogeneously distributed across the tidal flat. In this case, at algal concentrations between 0.68 and 1.80 g m −3 , the model predicts two alternative stable states: one with ample mussels that enhance sediment stabilization and experience a low mortality rate, the other a barren area without sediment stabilization and with high mortality rates preventing mussel establishment ( Fig. 3a ). When the algal concentration becomes too low (<0.68 g m −3 ), a tipping point occurs below which the mussel bed collapses to a barren state devoid of mussels, from which recovery is very difficult. Recovery only occurs when the algal concentration increases to sufficiently high levels (>1.80 g m −3 ), such that there is sufficient food for mussel beds to re-establish themselves, or when initial mussel density is sufficiently high to overcome the establishment-threshold. Hence, without self-organization, the model predicts an extensive range of environmental conditions where alternative stable states occur and where mussels beds are particularly vulnerable to tipping behaviour in response to disturbances. This model behaviour is qualitatively similar to that described by models of other ecosystems with alternative stable states, such as shallow lakes [28] , [29] . 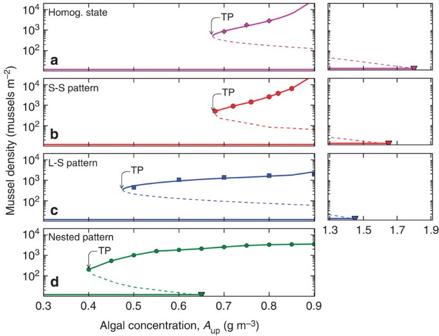Figure 3: Alternative stable states in mussel beds at different levels of spatial complexity. Bifurcation diagram representing the spatially averaged equilibrium density of mussel as a function of the algal concentration in the inflowing water (Aup), for four versions of the model: (a) without self-organization (that is, a homogeneous mussel bed); (b) with only small-scale self-organization generated through individual aggregation (S-S pattern); (c) with only large-scale self-organization generated by the interplay of competition and facilitation (L-S pattern); (d) with both forms of self-organization (nested pattern). TP indicates the tipping point. The dashed lines represent unstable equilibria, which act as a threshold below which the population will collapse. The solid lines of the upper equilibrium inaandcare obtained by integration of PDEs (equation (1)) via AUTO-07p using a one-dimensional space with a single peak, the solid lines inbanddare simple connections of the points derived by simulation, whereas all the points in these graphs are based on the IBM results. Note the slight deviance of the solid curves inaandcfrom the data points, which is due to noise created by variation in individual movement in the individual-based models. Figure 3: Alternative stable states in mussel beds at different levels of spatial complexity. Bifurcation diagram representing the spatially averaged equilibrium density of mussel as a function of the algal concentration in the inflowing water ( A up ), for four versions of the model: ( a ) without self-organization (that is, a homogeneous mussel bed); ( b ) with only small-scale self-organization generated through individual aggregation (S-S pattern); ( c ) with only large-scale self-organization generated by the interplay of competition and facilitation (L-S pattern); ( d ) with both forms of self-organization (nested pattern). TP indicates the tipping point. The dashed lines represent unstable equilibria, which act as a threshold below which the population will collapse. The solid lines of the upper equilibrium in a and c are obtained by integration of PDEs (equation (1)) via AUTO-07p using a one-dimensional space with a single peak, the solid lines in b and d are simple connections of the points derived by simulation, whereas all the points in these graphs are based on the IBM results. Note the slight deviance of the solid curves in a and c from the data points, which is due to noise created by variation in individual movement in the individual-based models. Full size image The combination of small-scale aggregative behaviour and large-scale ecosystem patterning strongly affects the functioning and resilience of mussel beds. First, mussel beds can survive at lower algal concentrations ( Fig. 3b–d ) and can persist at lower mussel densities ( Fig. 4a ) when small-scale or large-scale self-organization is introduced separately, but most strongly so when these processes are combined. The range of algal concentrations at which alternative stable states occur, and where the bed is vulnerable to disturbances, becomes only slightly smaller when either only small-scale or only large-scale self-organization is allowed, but is strongly reduced when both self-organizing processes are allowed to interact ( Fig. 4b ). Moreover, the combination of both small-scale and large-scale spatial self-organization leads to more rapid spatial pattern formation ( Fig. 4c ), and allows for a much faster recovery from external disturbances ( Fig. 4d ). This effect results from the fast aggregation of mussels in small-scale clusters, which lowers mortality and thereby increases local mussel density, thus facilitating the development of the large-scale banded patterns. Hence, small-scale aggregation allows the mussels to quickly overcome the establishment-threshold predicted by models without small-scale aggregation. These results demonstrate that the interaction between different levels of self-organization and the spatial complexity that emerges from this interaction can have striking effects on the stability, persistence and productivity of self-organized ecosystems. 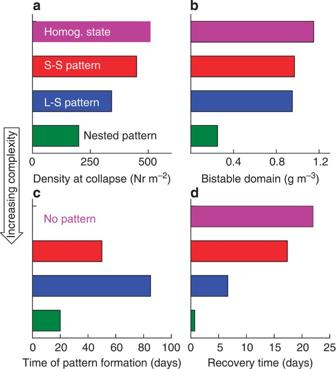Figure 4: Effects of increasing spatial complexity on ecosystem functioning. (a) Average mussel density at the tipping point (marked by down arrows inFig. 3, TP=tipping point). (b) Size of the bistable domain with respect to algal concentration. (c) Rate of pattern formation, which was calculated as the time required to reach stable spatial patterns when starting from a random initial distribution. (d) Recovery time after a large perturbation (30% reduction of mussel density). Each panel compares four model versions, where the colours indicate the types of patterns. Figure 4: Effects of increasing spatial complexity on ecosystem functioning. ( a ) Average mussel density at the tipping point (marked by down arrows in Fig. 3 , TP=tipping point). ( b ) Size of the bistable domain with respect to algal concentration. ( c ) Rate of pattern formation, which was calculated as the time required to reach stable spatial patterns when starting from a random initial distribution. ( d ) Recovery time after a large perturbation (30% reduction of mussel density). Each panel compares four model versions, where the colours indicate the types of patterns. Full size image Our results suggest that natural ecosystems may be much more resilient and less likely to experience catastrophic shifts when self-organization generates complexity at multiple spatial scales and organizational levels. Mussels beds on soft-bottom substrates are particularly interesting ecosystems in this respect, because different processes of self-organization rapidly create conspicuous regular spatial patterns at distinctly different scales, nested within one another. However, nested spatial patterns are not unique to mussel beds, and can also be observed in other ecosystems such as seagrass beds, coral reefs [7] and savannahs [9] ( Supplementary Data 1 ). Our study illustrates that in these systems, self-organizing processes driven by individual aggregation and spatial differentiation in growth rates may allow for enhanced persistence in the face of increasing stress, and faster recovery in the face of disturbances. The ever-increasing impact of human activities on natural landscapes (for example, by agricultural and urban development) often results in spatial homogenization of natural ecosystems, and restricts the movement and dispersal of many organisms [30] , [31] , [32] . This human influence may strongly impair self-organizing processes at multiple spatial scales and the resulting spatial complexity that is characteristic of many natural ecosystems. Our study demonstrates that this ‘spatial simplification’ can make populations and ecosystems more vulnerable to perturbation and increases the potential for catastrophic collapse to alternative and often degraded states. Allowing self-organization to generate patterns and complexity at multiple spatial scales may improve the intrinsic ability of ecosystems to withstand both natural and human-induced disturbances. The description of theoretical model To study how pattern formation at multiple spatial scales affects the resilience of mussel beds, we developed a model that combines a mathematical description of large-scale pattern formation in mussel beds [25] with an individual-based, numerical model for aggregative movement of mussels at small spatial scales [13] . In this model, large-scale population growth and losses processes are described by three partial differential equations, one describing changes in algal concentration in the benthic boundary layer A ( x, y, t ), one for mussel density on the bottom M ( x, y, t ) and one for sediment elevation S ( x, y, t ), each at location ( x, y ) and time t . Therefore, the model can be written as equation (1). We use the notation to represent mussel movement, which is modelled explicitly as random walks of individual mussels [13] . Statistical analysis of experimental movement trails revealed that the distances covered by the mussels during 1 min could be approximated by an exponential distribution [13] , [33] , where the frequency h of occurrence decreased with movement distance r ; h ( r , β )=(1/ β ) exp(− r / β ). Here, the scaling parameter β is a function of the densities of mussels in the neighbourhood. Statistical analysis of the relationship between movement speed and mussel density revealed that this scale parameter β is negatively affected by density at a scale of 1.5 cm, but positively affected by density at a scale of 6.0 cm. The scale-dependent feedback can be expressed as β =1/( p 0 + p 1 L 1 − p 2 L 2 ), where L 1 and L 2 represent the mussel densities at the two different scales, and the coefficients p 0 , p 1 and p 2 represent an intercept (movement speed at zero mussel density), and the coefficients of density dependence, respectively, which were all obtained from the regression analysis. Implementation of the model on a graphics processor For the PDE model, we used a spatial grid of 256 × 256 cells spanning a 50 × 50-metre area covering ~6 wavelengths ( Fig. 2d–f ), but 128 × 128 cells spanning a 20 × 20-metre area were used for the quantitative analysis of bifurcation analysis ( Fig. 3 ). Implementation of this model (1) consists of three steps. The first step is to calculate mussel growth and mortality, along with algal concentration and sediment elevation using the PDE components of the model (without mussel diffusion terms at here). The second step is to update local mussel density in the IBM representation of the mussels, using the new mussel densities predicted by the PDE. When the PDE predicts that mussel density decreases locally, a random selection of individual mussels is removed from the local grid cell of the IBM. When mussel density increases, new mussels are randomly added to the grid cell. The last step is to calculate mussel movement at the scale of the individual mussels. Experiments demonstrated that individual movement occurred at much faster time scales than ecosystem-level growth and mortality processes [13] , [20] . To facilitate the simulation process, we assumed a fixed factor of 33 between the two time scales. This simplification did not affect equilibrium densities. Owing to intensive calculations required to compute movement of all individual mussels, the simulation was implemented on a graphics processor, coded in the Compute Unified Device Architecture (CUDA) extension of the C language (NVIDIA-CUDA, https://developer.nvidia.com/cuda-gpus ) and computed on multiple NVIDIA Tesla C1060 high-performance computing boards. For sorting, we used the CUDA Data Parallel Primitives Library (CUDPP, http://cudpp.github.io). The model assumes a fixed (adult) mussel size, because even the high-performance computing boards that we used did not have sufficient computing power to describe the movement of large numbers of juvenile mussels. Each simulation run was started with a randomized distribution of mussels. The program code is available at ftp://public:public@dmgftp.nioz.nl/LiuCode/index.liu . Switching off small-scale and large-scale self-organization In the simulations we removed small-scale aggregative behaviour of the mussels by setting the exponential distribution to β =1/ p 0 . In this scenario, individual movement becomes random Brownian motion, that is, equivalent to standard diffusion, and hence can also be represented by the Laplace operator ▿ 2 M ( Supplementary Fig. 2 ). Simulation results suggest that the IBM model without small-scale aggregation accurately reproduces the self-organized spatial patterns predicted by the PDE model using a diffusion operator to describe mussel movement (see Supplementary Fig. 2 ). We removed large-scale ecosystem patterns by increasing the value of the diffusion coefficient of sediment to D s =0.005 m 2 h −1 , which is outside the domain allowing large-scale pattern formation (changing of the parameter, V or D m is possible [34] , [35] ). Finally, a completely homogeneous state was obtained by setting both individual mussel movement ( β ) and sediment diffusion ( D S ) to the above-mentioned values. We note that changing β and D s only affects movement processes. Hence mussel growth and mortality are not directly affected by changes in β and D s , only indirectly via the effect of β and D s on the formation of small-scale and large-scale patterns. This allows for identification of the emergent effects of pattern formation on the mean equilibrium values of A , M and S . Finally, a completely homogeneous state was obtained by setting both sediment diffusion and individual mussel movement to the above-mentioned values. Our analysis currently only investigates the sensitivity of the model to an increase in the algal concentration in the incoming water, A up . It is likely that the bifurcation analysis of Fig. 3 is sensitive to other critical parameters such as mussel mortality d m , its density dependence k m and other parameters. The high computing time required to analyse this model precludes such an analysis, although. We therefore based our analysis on estimates that are, for as much as possible, based on experiments in case of mussel movement, and literature evidence in case of growth and mortality processes. Moreover, we provide extensive bifurcation analyses of the models of small-scale and large-scale self-organization in previous papers [13] , [14] , [20] , [25] , [34] , [35] . Field photos of mussel patterns Field photos of mussel patterns with different spatial scales were taken on the tidal flats. Figure 2c was collected from the Gallow Point (53.245238N, −4.104166E) near Menai Bridge, UK, in July 2006, and Fig. 2a,b was collected from opposite to De Cocksdorp (53.159239 N, 4.890936 E) in Texel, The Netherlands, from August to September 2009. How to cite this article: Liu, Q.-X. et al. Pattern formation at multiple spatial scales drives the resilience of mussel bed ecosystems. Nat. Commun. 5:5234 doi: 10.1038/ncomms6234 (2014).